Pits confined in ultrathin cerium(IV) oxide for studying catalytic centers in carbon monoxide oxidation Finding ideal material models for studying the role of catalytic active sites remains a great challenge. Here we propose pits confined in an atomically thin sheet as a platform to evaluate carbon monoxide catalytic oxidation at various sites. The artificial three-atomic-layer thin cerium(IV) oxide sheet with approximately 20% pits occupancy possesses abundant pit-surrounding cerium sites having average coordination numbers of 4.6 as revealed by X-ray absorption spectroscopy. Density-functional calculations disclose that the four- and five-fold coordinated pit-surrounding cerium sites assume their respective role in carbon monoxide adsorption and oxygen activation, which lowers the activation barrier and avoids catalytic poisoning. Moreover, the presence of coordination-unsaturated cerium sites increases the carrier density and facilitates carbon monoxide diffusion along the two-dimensional conducting channels of surface pits. The atomically thin sheet with surface-confined pits exhibits lower apparent activation energy than the bulk material (61.7 versus 122.9 kJ mol −1 ), leading to reduced conversion temperature and enhanced carbon monoxide catalytic ability. Catalysis can accelerate the speed of chemical reactions through changing the reaction pathway and lowering the activation energy, hence its wide application in diverse fields such as industrial ammonia production in Haber process [1] , the catalytic converters in automobiles [2] and the enzymatic catalytic processes in living systems [3] . According to the basic theory originally proposed by Taylor, in gas-phase catalytic systems [4] , catalytic reactions usually occur at the active sites of catalysts, for which the crystalline defects such as step edges and kink sites with low coordination numbers are the favourable catalytic reaction centres [5] , [6] , [7] , [8] . Heterogeneous processes, generally consist of three consecutive steps of adsorption, chemical reaction and desorption, and the corresponding catalytic rate is often limited by one elementary step, referred to the rate-determining step [8] , [9] . Taking the extensively studied catalytic CO oxidation as an example, the catalytic reaction rate is typically limited by the adsorption and dissociation of O 2 molecules on the active sites of catalysts [10] . Up to now, various reaction mechanisms for CO oxidation have been proposed, among which the three most popular mechanisms are the Langmuir-Hinshelwood mechanism [8] , [11] , [12] , the Eley-Rideal mechanism [8] , [13] and the Mars-van Krevelen mechanism [14] . Although these mechanisms have been proposed to investigate the catalytic reaction processes, atomic-level insights into the underlying mechanism of catalysis are less explored. This is mainly due to the large differences between idealized models and real catalysts, and hence the knowledge gained from these models is not readily applicable to real catalysts. To evaluate where catalysis occurs and which site has the highest activity, simplifying and bridging the catalyst model with the real catalyst is of paramount importance. Recently, for better understanding the fundamental mechanism in catalytic CO oxidation, reactions on oriented crystals with a predominantly exposed facet have been further explored [15] , [16] , [17] , [18] , [19] , [20] , [21] , [22] , [23] , thanks to the single active site on these facets. For instance, theoretical calculations revealed that CO had stronger chemisorption on the {110} and {100} facets of CeO 2 than on the {111} facets [17] , [18] . This has been experimentally demonstrated by the fact that the rod-like CeO 2 exposing {110} and {100} facets showed obviously improved CO catalytic properties than octahedron-like CeO 2 exposing {111} facets [19] . Also, Xie et al. [20] observed that the cube-like CeO 2 crystals with exposed {100} facets exhibited superior CO oxidation properties than the truncated octahedron-like CeO 2 crystals with exposed {100} and {111} facets. Although the unique crystal plane has provided a good platform for understanding the role of active sites in catalysis, the relatively low ratio of surface active sites to the total atom numbers makes the quantification of a model-performance relationship a great challenge ( Fig. 1a ). Fortunately, recent studies have revealed that nanoscale crystallites such as CeO 2 nanostructures are beneficial to the CO oxidation reaction thanks to their downsizing effect [24] , [25] , [26] , [27] , [28] , [29] . For example, Botana et al. [25] have found that CeO 2 nanotubes exhibited 400-fold higher CO oxidation compared to polycrystalline CeO 2 powder owing to their superior redox properties. Also, Tsang et al. have demonstrated that the quantum size effect could enable the nanosize CeO 2 (below 5 nm) to possess dramatically increased surface superoxide species [30] , which undoubtedly contributed to improve the catalytic oxidation activity [30] , [31] , [32] . In addition, Cormatt et al. have illustrated that nanocrystalline CeO 2 could increase the activity of Au for CO oxidation by two orders of magnitude through effectively adsorbing and activating O 2 molecules [24] . These results indicated that nanoscale size effects could provide more active sites and hence helped to improve the catalytic properties [33] , [34] . Hence, developing a material model with exposed unique crystal plane as well as nanoscale thickness holds the key to disclosing the role of active sites in catalysis. 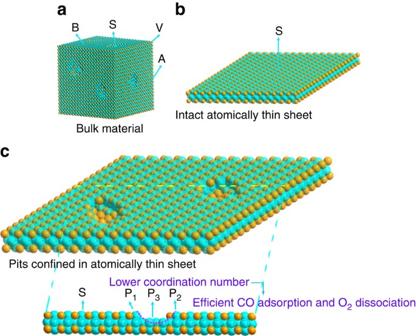Figure 1: Schematic illustration for evaluating catalysis location and activity. (a) Bulk CeO2; (b) intact and (c) atomically thin CeO2sheets with surface-confined pits; P1and P2stand for the representative pit-surrounding surface Ce sites, while P3represents the bottom Ce site of the pit; S stands for the surface Ce site of atomically thin sheet and around the defects of bulk material; A, V and B represent the arris, vertex and surface Ce sites of bulk material, respectively. Figure 1: Schematic illustration for evaluating catalysis location and activity. ( a ) Bulk CeO 2 ; ( b ) intact and ( c ) atomically thin CeO 2 sheets with surface-confined pits; P 1 and P 2 stand for the representative pit-surrounding surface Ce sites, while P 3 represents the bottom Ce site of the pit; S stands for the surface Ce site of atomically thin sheet and around the defects of bulk material; A, V and B represent the arris, vertex and surface Ce sites of bulk material, respectively. Full size image In this work, taking the typical CO oxidation catalyst of CeO 2 as an example, an ideal model consisting of intact atomically thin CeO 2 sheets is developed to maximize the number of coordinately unsaturated active sites, as shown in Fig. 1b . Due to the atomic thickness and specific surface area, such sheets possess the features of relatively disperse active sites and a high ratio of surface active sites to the total atom numbers. To further promote the activity of the catalytic sites, we can make lots of artificial pits with lower coordination numbers on the surface of atomically thin CeO 2 sheets ( Fig. 1c ). To date, it remains particularly challenging to synthesize atomically thin CeO 2 sheets with surface-confined pits in a controllable manner, due to the difficulty in bond-cleavage and the absence of an intrinsic driving force for the formation of coordinatively unsaturated active sites [7] , [8] . To meet this challenge, we herein develop an ‘ultrafast open space transformation’ strategy and successfully synthesize three-atom-layer thin CeO 2 sheets with ~20% pits occupancy. X-ray absorption fine structure spectroscopy (XAFS) and density-functional calculations (DFT) disclose that the pit-surrounding Ce sites with average Ce-O coordination numbers as low as 4.6 serve as the catalytically active centres. These centres play essential roles in O 2 activation, CO adsorption and diffusion, which lead to decreased apparent activation energy from 122.9 to 61.7 kJ mol −1 as well as obviously reduced CO conversion temperatures. This study provides valuable insights into the role of active centres in catalysis through a semi-quantitative model-structure-performance relationship, holding great promise for designing catalysts with highly efficient active centres. Characterization of ultrathin CeO 2 sheets with surface pits As depicted in Fig. 2a and Supplementary Fig. S1 , the successful synthesis of ultrathin CeO 2 sheets took advantage of an intermediate precursor of ultrathin CeCO 3 OH sheets. During the formation of this precursor, the peculiar arrangement of oleate ions around the surface of Ce 3+ played a vital role: Ce 3+ initially interacted with oleate ions to form Ce-oleate complexes via an electrostatic interaction and hence assembled into atomically thin two-dimensional structure driven by the hydrophobic effect of oleate tails [35] . After addition of NH 3 ·H 2 O followed by hydrothermal treatment for 48 h, the ultrathin CeCO 3 OH sheets were obtained and fully characterized in Supplementary Fig. S2 . And then, direct heating of the precursor at 400 °C for 2 min in air not only resulted in the formation of clean three-atom-layer thin CeO 2 sheets, but also brought on numerous pits on their surfaces ( Fig. 2b–d and Supplementary Figs S3–S5 ). The high-resolution transmission electron microscopy (TEM) image in Fig. 2b clearly revealed the high [110] orientation of the CeO 2 sheets, while the atomic force microscopy (AFM) image and the corresponding height profile in Fig. 2c,d showed their height of about 0.60 nm, which fairly agreed with the 0.57 nm thickness of three-atom-thin CeO 2 slab along the [110] direction. More importantly, the HRTEM and AFM images in Fig. 2b–d also depicted that the pits possessed an occupancy of about 20% in the three-atom-thick CeO 2 sheets, indicating the presence of abundant pit-surrounding Ce sites. By contrast, the heating at higher temperature of 550 °C with a shorter time of 10 s only resulted in the formation of clean three-atom-thick CeO 2 sheets without surface pits ( Fig. 2a and Supplementary Fig. S6 ), strongly suggesting that the heating temperature and time played an important role in the formation of pits on the surfaces of ultrathin CeO 2 sheets ( Supplementary Figs S7–S9 ). 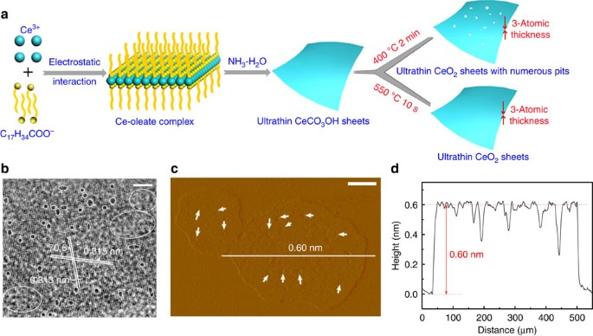Figure 2: Formation process and characterization of the ultrathin CeO2sheets with numerous surface pits. (a) Schematic illustration for the formation of ultrathin CeO2sheets with numerous surface pits and intact ultrathin CeO2sheets. Note that the heating temperature and time have a vital role in the formation of pits on their surface. (b–d) Characterizations for the three-atom-thin CeO2sheets with numerous surface pits: (b) HRTEM image, (c) AFM image and (d) the height profile along the white line indicated in (c). The scale bars in (c) and (d) are 3 and 100 nm, respectively. The inset circles and arrows in (b) and (c) denote the presence of pits on their surface. Figure 2: Formation process and characterization of the ultrathin CeO 2 sheets with numerous surface pits. ( a ) Schematic illustration for the formation of ultrathin CeO 2 sheets with numerous surface pits and intact ultrathin CeO 2 sheets. Note that the heating temperature and time have a vital role in the formation of pits on their surface. ( b – d ) Characterizations for the three-atom-thin CeO 2 sheets with numerous surface pits: ( b ) HRTEM image, ( c ) AFM image and ( d ) the height profile along the white line indicated in ( c ). The scale bars in ( c ) and ( d ) are 3 and 100 nm, respectively. The inset circles and arrows in ( b ) and ( c ) denote the presence of pits on their surface. Full size image Synchrotron radiation XAFS measurements To obtain quantitative structural parameters around the pits of the three-atom-thick CeO 2 sheets, XAFS measurements at Ce L 3 -edge were carried out at the U7C beamline of the National Synchrotron Radiation Laboratory, China. As shown in Fig. 3a , the Ce L 3 -edge k 2 χ( k ) oscillation curve for the ultrathin CeO 2 sheets with numerous surface pits displayed obvious differences compared with the ultrathin CeO 2 sheets and bulk CeO 2 ( Supplementary Fig. S10 ). This was further verified by their corresponding Fourier transformed (FT) k 2 χ( k ) functions in Fig. 3b , which displayed that the two main peaks gradually shifted to the low R direction along with obviously decreased intensities, qualitatively revealing their distinct local atomic arrangement. Moreover, to achieve quantitative structural parameters around Ce atoms, a least-squares curve fitting was conducted and the details of the EXAFS data fitting are provided in the Methods section. As for the ultrathin CeO 2 sheets, Table 1 revealed that the distances and coordination numbers for Ce-O, Ce-Ce, Ce-O-O and Ce-Ce-O coordinations reduced remarkably, while their disorder degrees increased significantly as compared with bulk counterpart, suggesting a noticeable distortion on their surface. Importantly, the pit-surrounding Ce-O distances, confined in the ultrathin CeO 2 sheets with numerous surface pits, were contracted from 2.327 to 2.302 Å, and their coordination numbers remarkably decreased from 6.5 to 4.6, associated with significantly increased disorder degrees relative to the ultrathin CeO 2 sheets ( Table 1 ). This implied an obvious distortion surrounding the pits of ultrathin CeO 2 sheets. Notably, such surface distortion has already been observed in previously reported atomically thin two-dimensional sheets and has also been demonstrated to endow them with excellent structural stability and increased states density [6] , [7] , [36] . As depicted by the calculated densities of states in Fig. 3c , the presence of abundant coordination-unsaturated pit-surrounding Ce sites in the ultrathin CeO 2 sheets led to the formation of defect states near the Fermi level, which resulted in an obvious increase of hole carrier concentration with respect to the ultrathin CeO 2 sheets and bulk counterpart [37] . As will be shown, these features enabled the ultrathin CeO 2 sheets with numerous surface pits to realize fast CO diffusion along the two-dimensional conducting channel of surface pits and hence improved their CO catalytic properties [6] , [7] , [38] . 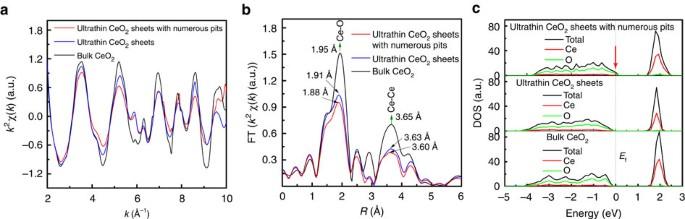Figure 3: Synchrotron radiation XAFS measurements. (a) CeL3-edge extended XAFS oscillation functionk2χ(k), (b) the corresponding Fourier transforms FT (k2χ(k)), (c) the calculated densities of states for the ultrathin CeO2sheets with numerous surface pits, ultrathin CeO2sheets and bulk CeO2, respectively. a.u., arbitrary unit. Figure 3: Synchrotron radiation XAFS measurements. ( a ) Ce L 3 -edge extended XAFS oscillation function k 2 χ( k ), ( b ) the corresponding Fourier transforms FT ( k 2 χ( k )), ( c ) the calculated densities of states for the ultrathin CeO 2 sheets with numerous surface pits, ultrathin CeO 2 sheets and bulk CeO 2 , respectively. a.u., arbitrary unit. Full size image Table 1 EXAFS curve-fitting results. Full size table Catalytic carbon monoxide oxidation Summarizing the above XAFS, TEM and AFM results, an ideal model for three-atom-thick CeO 2 sheets with surface-confined pits is built to gain atomic-level insights into the underlying catalytic mechanism ( Fig. 4c ). According to the widely accepted Langmuir-Hinshelwood mechanism [8] , [11] , [12] , the CO oxidation occurring on the pit-surrounding Ce sites may consist of the following elementary steps: (1) Adsorption of CO and O 2 molecules from the gas phase onto the pit-surrounding Ce sites; (2) dissociation of O 2 molecules on the pit-surrounding Ce sites; (3) reaction between CO and dissociated O atom to form CO 2 ; (4) desorption of CO 2 to the gas phase. In addition, it is noticeable that CO should diffuse to the nearby atomic O before their reaction to form CO 2 , in which the CO molecules need to overcome a diffusion barrier [39] , [40] . DFT calculations were performed on various pit-surrounding Ce sites and on-surface Ce sites in order to identify the active sites. 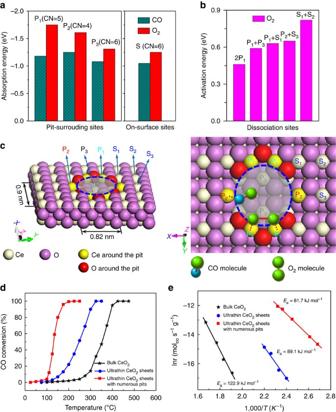Figure 4: Catalytic carbon monoxide oxidation. (a) Calculated adsorption energies for CO and O2molecules on the pit-surrounding Ce sites (P1~P3) and on-surface Ce sites (S1~S3), and (b) calculated activation energies for O2dissociation on the adjacent Ce sites of ultrathin CeO2sheets with numerous pits; the coordination numbers of P1, P2, P3, S1, S2and S3are 5, 4, 6, 6, 6 and 6, respectively. (c) Overhead and top views of schematic structures for the three-atom-thick CeO2sheets with a pit size of 0.90 nm × 0.82 nm (This size is fairly consistent with that statistically calculated from the HRTEM image inFig. 2b); the CO molecules prefer to adsorb at P2site, while the O2molecules tend to adsorb and dissociate at the adjacent P1sites. (d) Catalytic activity for CO oxidation versus reaction temperatures (experimental error: ±3%) and (e) the corresponding Arrhenius plot for the three CeO2samples (experimental error: ±3%). Figure 4a clearly revealed that CO and O 2 molecules exhibited the highest adsorptive energies (absolute values) at pit-surrounding 4-coordinated Ce site (P 2 , −1.25 eV) and 5-coordinated Ce site (P 1 , −1.75 eV), respectively. This indicated that the CO and O 2 molecules preferred to adsorb at the pit-surrounding Ce sites with different coordination numbers and hence would not block the active sites for each other, thus effectively avoiding the catalyst poisoning. Also, the dissociation of O 2 molecules needed the lowest activation energy of 0.46 eV at the two adjacent 5-coordinated Ce sites (2P 1 , Fig. 4b ), suggesting that they preferably dissociated into oxygen atoms on the dual adjacent fivefold coordinated Ce sites and their corresponding transition state was shown in Fig. 4c . Considering the relatively small energy barrier of 0.12 eV for the CO+O associative desorption, it was suggested that the bonding strength for O atoms at the pit-surrounding Ce sites was optimum and would make these sites active [5] . The above results revealed that the coordination number and spatial distribution of the pit-surrounding Ce sites played a crucial role in CO catalytic oxidation. In this case, the pits with different size and shape would theoretically achieve the similar CO adsorption energies and O 2 activation energies when their pits could provide the 4- and 5-coordinated pit-surrounding Ce sites with similar percentage and spatial distribution ( Supplementary Fig. S11 ). Moreover, the CO diffusion barriers on the pit-surrounding Ce sites and on-surface Ce sites were calculated to be 0.08 and 0.17 eV, respectively. The lowered CO diffusion barrier on the pit-surrounding Ce sites could be benefited from their increased states density near the Fermi level ( Fig. 3c ) and hence contributed to lower the overall activation energy, thus finally improving their CO oxidation activity. In this case, the adsorbed CO molecules at 4-coordinated Ce site could effectively diffuse into the 5-coordinated Ce site along the two-dimensional conducting channel of surface pits and hence reacted with the dissociated oxygen atoms to produce CO 2 . Thus, although it was difficult to distinguish the rate-determining step and accurately evaluate the overall activation energy without full kinetic simulations, the simple analysis of the above activation energies helped to draw the following conclusions: (1) The step of O 2 activation was the rate-limiting step for the ultrathin CeO 2 sheets with numerous surface pits, since the calculated O 2 activation energy of ~0.46 eV on the pit-surrounding Ce sites was much higher than the corresponding calculated CO+O associative desorption energy (0.12 eV) and the CO diffusion energy (0.08 eV); (2) the overall activation energy on the pit-surrounding Ce sites could be roughly evaluated to be the value between 0.46 and 0.66 eV (corresponding to the range from 44.4 to 63.6 kJ mol −1 ), fairly consistent with their apparent activation energy of 61.7 kJ mol −1 in Fig. 4e . Based on the above results, one could conclude that the ultrathin CeO 2 sheets with numerous surface pits had ~20% pits occupancy, in which the abundant pit-surrounding Ce sites served as the active sites in CO catalytic oxidation and such a large amount of highly active pit-surrounding Ce sites could in fact support them to quickly complete the CO catalytic oxidation at a low reaction temperature ( Fig. 4d ). By contrast, for the intact ultrathin CeO 2 sheets without surface pits and bulk counterpart ( Supplementary Figs S6 and S10 ), only the surface Ce atoms could serve as the active sites to catalyse CO oxidation. Note that the pit-surrounding Ce site has an average coordination number of 4.6, much smaller than that (6.5) of the surface Ce site in the ultrathin CeO 2 sheets ( Fig. 3 ), reasonably exhibiting higher catalytic activity than that at the on-surface Ce site. The conclusion could be further confirmed by their corresponding adsorption energies for CO and O 2 molecules as well as O 2 dissociation energies in Fig 4a,b . In this case, the ultrathin CeO 2 sheets with numerous surface pits could theoretically possess lowered overall activation energy as well as accelerated catalytic reaction rate compared with the ultrathin CeO 2 sheets without surface pits and the bulk counterpart. Figure 4: Catalytic carbon monoxide oxidation. ( a ) Calculated adsorption energies for CO and O 2 molecules on the pit-surrounding Ce sites (P 1 ~P 3 ) and on-surface Ce sites (S 1 ~S 3 ), and ( b ) calculated activation energies for O 2 dissociation on the adjacent Ce sites of ultrathin CeO 2 sheets with numerous pits; the coordination numbers of P 1 , P 2 , P 3 , S 1 , S 2 and S 3 are 5, 4, 6, 6, 6 and 6, respectively. ( c ) Overhead and top views of schematic structures for the three-atom-thick CeO 2 sheets with a pit size of 0.90 nm × 0.82 nm (This size is fairly consistent with that statistically calculated from the HRTEM image in Fig. 2b ); the CO molecules prefer to adsorb at P 2 site, while the O 2 molecules tend to adsorb and dissociate at the adjacent P 1 sites. ( d ) Catalytic activity for CO oxidation versus reaction temperatures (experimental error: ±3%) and ( e ) the corresponding Arrhenius plot for the three CeO 2 samples (experimental error: ±3%). Full size image To verify the predictions from the above theoretical model, the corresponding CO catalytic properties of the ultrathin CeO 2 sheets with numerous surface pits were investigated. As shown in Fig. 4d , they possessed 50% CO conversion at 131 °C, which was 117 °C and 223 °C lower than that of the ultrathin CeO 2 sheets and bulk counterpart, respectively. At the same temperature of 131 °C, the ultrathin CeO 2 sheets and bulk CeO 2 only showed CO conversion ratio of 3.2 and 0.89%, over 15 and 50 times smaller than that of the ultrathin CeO 2 sheets with numerous surface pits. Also, the complete CO conversion temperature for the ultrathin CeO 2 sheets with numerous surface pits was about 200 °C, strikingly lower than that of the ultrathin CeO 2 sheets (325 °C) and bulk counterpart (425 °C). To the best of our knowledge, the half conversion temperature for the ultrathin CeO 2 sheets with numerous surface pits was much lower than all of those reported values for parent CeO 2 (refs 41 , 42 , 43 , 44 ), strongly suggesting the remarkably improved low-temperature CO catalytic activity. Moreover, the Arrhenius plot in Fig. 4e revealed that the apparent activation energy for the ultrathin CeO 2 sheets with numerous surface pits was 61.7 kJ mol −1 , obviously smaller than the values of 89.1 and 122.9 kJ mol −1 for the ultrathin CeO 2 sheets and bulk counterpart. This implied that the CO oxidation catalysed by the ultrathin CeO 2 sheets with numerous surface pits involved different catalytically active sites in comparison with the other two CeO 2 samples [45] , in which the 4-coordinated and 5-coordinated pit-surrounding Ce sites undoubtedly accounted for the eminently lowered apparent activation energy and subsequently decreased CO conversion temperatures. Accordingly, the obviously promoted CO catalytic performances for ultrathin CeO 2 sheets with numerous surface pits were fairly consistent with the corresponding theoretical model predictions, providing strong evidence for the validity and reliability of the designed model. Of note, as shown in Supplementary Fig. S12 , one can conclude that the ultrathin CeO 2 sheets with surface-confined pits possessed two types of active sites including very active pit-surrounding Ce atoms and less active surface Ce atoms: when the surface pits had a low percentage such as 2% ( Supplementary Fig. S7 ), the small amount of pit-surrounding Ce atoms and other surface Ce atoms could together act as the active sites to catalyse the CO oxidation reactions; whereas, when the pits occupancy in the ultrathin CeO 2 sheets was up to 10%, the pit-surrounding Ce atoms could serve as the preferentially active sites to support them quickly to complete the CO oxidation reaction in a narrow temperature range ( Supplementary Fig. S9 ). As is well-known, the auto-ignition temperature of CO molecules is as high as 608.89 °C. After adding a catalyst such as bulk CeO 2 , the ignition temperature corresponding to 10% CO conversion could be reduced to 281 °C ( Fig. 4d ), verifying that the catalyst could indeed increase the reaction rate for CO oxidation. More interestingly, our designed three-atom-thick CeO 2 sheets with surface-confined pits further lowered the ignition temperature down to 106 °C. This raises important questions: what causes the strikingly different catalytic activity in the same catalyst material? How does it function? It is noticeable that the catalysis usually occurs at the active sites and the different active sites often lead to distinct CO catalytic reactivities [15] , [30] , [46] , [47] . Here, DFT calculations in Fig. 4a,b revealed that the pit-surrounding Ce sites confined in atomically thin sheets were identified as the most favourable active centres for CO catalytic oxidation. In addition, the XAFS results in Table 1 showed that the active centres possessed the average coordination numbers of 4.6, which was much lower than that of other various active sites. Thus, it was the peculiar active centres with lower coordination numbers that brought about the enhanced CO oxidation. In the active centres, the 4- and 5-coordinated pit-surrounding Ce sites favoured for CO adsorption and O 2 activation, respectively, which effectively decreased the catalyst poisoning chance. Also, the highly coordination-unsaturated pit-surrounding Ce sites resulted in the increased carrier density near the Fermi level ( Fig. 3c ), which ensured fast CO diffusion along the two-dimensional conducting channel of surface pits and subsequently facilitated CO oxidation by the dissociated O atoms [6] , [7] , [32] , [48] . In other words, the active centres consisting of pit-surrounding Ce sites were beneficial to O 2 activation, CO adsorption and diffusion. In addition, the extremely high fraction of surface Ce atoms as well as the quantum size effect in the ultrathin CeO 2 sheets could also contribute to lower their overall activation energy and definitely accelerate the speed of CO catalytic reaction compared with the bulk counterpart [24] , [25] , [26] , [27] , [28] , [29] , [30] , [31] , [32] , which could be verified by the CO conversion curves and the corresponding activation energies of the intact ultrathin CeO 2 sheets and bulk counterpart in Fig. 4d,e . As such, the different activation energies between the ultrathin CeO 2 sheets with numerous surface pits and the bulk counterpart were not only due to the presence of surface pits but also due to the quantum effects at the nano-size. That is to say, in the ultrathin CeO 2 sheets with numerous surface pits, the quantum size effect and the abundant highly active pit-surrounding Ce sites could contribute to lower their overall activation energy and definitely increase the speed of CO catalytic reaction. Actually, the experimental results in Fig. 4d,e showed that the apparent activation energy for the ultrathin CeO 2 sheets with numerous surface pits remarkably decreased from 122.9 to 61.7 kJ mol −1 , and the corresponding CO conversion temperatures also reduced dramatically as compared to the bulk counterpart, verifying the predictions of the theoretical model. As a consequence, we bridged the gap between theoretical model and real catalyst, and subsequently identified the catalytically active centre through semi-quantifying the model-structure-performance relationship, which deepened our understanding about the underlying nature of catalysis. In conclusion, conceptually new atomically thin sheets with surface-confined pits were proposed as an excellent platform to study the role of active sites in catalysis. Freestanding three-atom-thick CeO 2 sheets with ~20% surface pits occupancy were synthesized via an ‘ultrafast open space transformation’ strategy and taken as an example to semi-quantify the model-structure-performance relationship. XAFS results directly evidenced the lower average coordination number of 4.6 for the abundant pit-surrounding Ce sites, which in fact served as the catalytically active centres. DFT calculations demonstrated that the 4- and 5-coordinated pit-surrounding Ce sites performed their respective functions in CO adsorption and O 2 activation, thus reducing the activation barrier and decreasing the catalyst poisoning chance. Also, the highly coordination-unsaturated pit-surrounding Ce sites brought about the increased hole carrier density and hence assured fast CO diffusion along the two-dimensional conducting channel of surface pits. As a result, the atomically thin CeO 2 sheets with surface-confined pits lowered the apparent activation energy from 122.9 to 61.7 kJ mol −1 and definitely decreased the CO conversion temperatures. This work provides crucial insights into the role of active centres in catalysis through first semi-quantifying the model-structure-performance relationship, opening the door for designing catalytic centres. Synthesis details Synthesis of freestanding ultrathin CeCO 3 OH sheets: 1.5 mmol sodium oleate was initially dissolved in 20 ml distilled water. Then, 1 mmol CeCl 3 ·6H 2 O was dissolved in 10 ml distilled water and injected to the above solution followed by vigorous stirring for 30 min. After adding 9 ml NH 3 ·H 2 O dropwise to the above solution and stirring for 1 h, the mixture was transferred into a 50 ml Teflon-lined autoclave, sealed and heated at 180 °C for 48 h. The system was then allowed to cool down to room temperature naturally, the final product was collected by centrifuging the mixture, washed with cyclohexane for many times and then dried in vacuum overnight for further characterization. Synthesis of freestanding ultrathin CeO 2 sheets with numerous surface pits: the as-obtained white ultrathin CeCO 3 OH sheets were directly heated at 400 °C for 2 min in air and then cooled to room temperature. The brilliant yellow powders were collected for further characterization. Synthesis of freestanding intact ultrathin CeO 2 sheets: the as-obtained white ultrathin CeCO 3 OH sheets were directly heated at 550 °C for 10 s in air and then cooled to room temperature. The brilliant yellow powders were collected for further characterization. Characterization XRD patterns were recorded by using a Philips X’Pert Pro Super diffractometer with Cu Kα radiation (λ=1.54178 Å). TEM images and high-resolution TEM image were performed by using a JEOL-2010 TEM with an acceleration voltage of 200 kV. The field emission scanning electron microscopy images were performed by using a FEI Sirion-200 SEM. AFM study in the present work was performed by means of Veeco DI Nano-scope MultiMode V system. X-ray photoelectron spectra (XPS) were acquired on an ESCALAB MKII with Mg Kα (h υ =1253.6 eV) as the excitation source. The binding energies obtained in the XPS spectral analysis were corrected for specimen charging by referencing C 1 s to 284.5 eV. The IR spectra were measured on a NICOLET FT-IR spectrometer, using pressed KBr tablets. Raman spectra were detected by a RenishawRM3000 Micro-Raman system. Thermal gravimetric analysis of the as-synthesized samples was carried out on a Shimadzu TA-50 thermal analyser at a heating rate of 10 °C min −1 from room temperature to 800 °C. The Ce L 3 -edge XAFS was measured at the 1W1B beamline of Beijing Synchrotron Radiation Factory (BSRF) and the U7C beamline of the National Synchrotron Radiation Laboratory, China. The storage ring of the BSRF was operated at 2.5 GeV with a maximum current of 250 mA, and National Synchrotron Radiation Laboratory was operated with a storage ring working at the energy of 800 MeV and a maximum electron current of 300 mA. EXAFS data fitting Note that the HRTEM result in Fig. 2b clearly reveals that the pits possess an occupancy of about 20% in the ultrathin CeO 2 sheets with numerous surface pits. As such, 20% Ce-O distances and coordination numbers surrounding the pits of the ultrathin CeO 2 sheets are regarded to be shrunk during their EXAFS curve-fitting, while the other 80% Ce-O distances and coordination numbers still remain the same as that of intact ultrathin CeO 2 sheets without surface pits. As shown in Fig. 3b , the FT curve of bulk CeO 2 exhibited two main peaks at 1.95 and 3.65 Å, corresponding to the nearest Ce-O and next nearest Ce-Ce coordinations, respectively. For the ultrathin CeO 2 sheets, the Ce-O and Ce-Ce peak position exhibited a noticeable shift to 1.91 and 3.63 Å, associated with obvious reduction in their peak intensities. Contrastingly, for the ultrathin CeO 2 sheets with numerous surface pits, the intensities of these two peaks further decreased significantly, and most importantly, the Ce-O and Ce-Ce peaks were further shifted to 1.88 and 3.60 Å, qualitatively revealing their different local atomic arrangement compared with ultrathin CeO 2 sheets and bulk counterpart. Moreover, to achieve quantitative structural parameters around Ce atoms in the ultrathin CeO 2 sheets with numerous surface pits, a least-squares curve parameter fitting for the Ce-O, Ce-Ce, Ce-O-O and Ce-Ce-O peaks was conducted. The fitting results for the ultrathin CeO 2 sheets in Table 1 revealed that the distances and coordination numbers for the Ce-O, Ce-Ce, Ce-O-O and Ce-Ce-O coordinations reduced remarkably, while their disorder degrees increased significantly compared with bulk counterpart, suggesting a noticeable distortion on their surface. By contrast, the ultrathin CeO 2 sheets with numerous surface pits possessed further contracted distances and decreased coordination numbers for the Ce-O, Ce-Ce, Ce-O-O and Ce-Ce-O coordinations, along with further increased disorder degrees. Especially, the Ce-O distances surrounding the pits of the ultrathin CeO 2 sheets were obviously contracted from 2.327 to 2.302 Å, and their coordination numbers remarkably decreased from 6.5 to 4.6, associated with significantly increased disorder degrees compared to the ultrathin CeO 2 sheets. Calculation details Our first-principles density functional theory (DFT) calculations were performed using a plane wave basis set with the projector augmented plane-wave method [46] , [47] , [48] , [49] . The exchange-correlation interaction is described within the generalized gradient approximation [50] , [51] . The energy cutoff is set to 400 eV, and the atomic positions are allowed to relax until the energy and force are less than 10 −4 eV and 5 × 10 −3 eV Å −1 , respectively. The ultrathin CeO 2 sheets with numerous surface pits were simulated by periodically repeating the CeO layers along the [110] direction of the unit cell. Each sheet model consists of three CeO planes and is separated by a vacuum region of 15 Å. An elliptical void area by removing partial surface Ce and O atoms on the ultrathin sheet was used to simulate the pit. For the ultrathin CeO 2 sheets, they were simulated by periodically repeating the CeO layers along the [110] direction of the unit cell. Each sheet model consists of three CeO planes and is separated by a vacuum region of 15 Å. The comparison calculations for bulk CeO 2 were performed within supercells constructed from a standard unit cell of CeO 2 lattice. Moreover, we calculated the adsorption energy of CO and O 2 molecules surrounding the pits for various-sized pit models. The adsorption energy ΔE ads is defined as follows: where E tot (NS+AD), E tot (NS) and E tot (AD) are the total energies of CO and/or O 2 molecule adsorbing on the ultrathin CeO 2 sheet with numerous surface pits, the ultrathin CeO 2 sheet with numerous surface pits, and the adsorbent CO/O 2 molecules, respectively. The negative value of ΔE ads implies that adsorption is exothermic, so more the negative value of the ΔE ads , more is the stability of the model. Furthermore, the activation barriers of O 2 dissociation were calculated by the climbing image nudged elastic band method [52] , [53] , in which the zero energy reference is O 2 in gas phase. Catalytic activity measurements The catalytic properties of CO oxidation for CeO 2 were conducted in a quartz-tube plug flow reactor using 50 mg catalyst in a mixed gas of 1 vol% CO and 99 vol% dried air at a flow rate of 40 ml min −1 corresponding to a gas hourly space velocity of 48,000 ml h −1 g −1 . The catalyst was heated to the desired temperatures at a rate of 2 °C min −1 and then kept for 30 min until the catalytic reaction reached a steady state. Then, the composition of effluent gas was analysed by a portable intelligent professional CO 2 detector (Keernuo Gt901, Shenzhen Keernuo Technology Co. Ltd). The CO conversion was calculated from the change in CO 2 concentration of the inlet and outlet gases. Each experiment for the CO conversion was repeated at least three times to ensure reproducibility and to assess the range of experimental errors associated with the experiments, and the experimental error was assessed to be within±3.0%. How to cite this article: Sun, Y. et al. Pits confined in ultrathin cerium(IV) oxide for studying catalytic centres in carbon monoxide oxidation. Nat. Commun. 4:2899 doi: 10.1038/ncomms3899 (2013).